Vocalization frequency and duration are coded in separate hindbrain nuclei Temporal patterning is an essential feature of neural networks producing precisely timed behaviours such as vocalizations that are widely used in vertebrate social communication. Here we show that intrinsic and network properties of separate hindbrain neuronal populations encode the natural call attributes of frequency and duration in vocal fish. Intracellular structure/function analyses indicate that call duration is encoded by a sustained membrane depolarization in vocal prepacemaker neurons that innervate downstream pacemaker neurons. Pacemaker neurons, in turn, encode call frequency by rhythmic, ultrafast oscillations in their membrane potential. Pharmacological manipulations show prepacemaker activity to be independent of pacemaker function, thus accounting for natural variation in duration which is the predominant feature distinguishing call types. Prepacemaker neurons also innervate key hindbrain auditory nuclei thereby effectively serving as a call-duration corollary discharge. We propose that premotor compartmentalization of neurons coding distinct acoustic attributes is a fundamental trait of hindbrain vocal pattern generators among vertebrates. Neural networks provide exact timing of motor neuron activity for temporally precise behaviours [1] , [2] , [3] . Most recent studies of central mechanisms of vocalization, including those for speech, focus on forebrain circuits with insights mainly coming from brain-imaging studies and local field potential recordings in humans [4] , [5] , [6] , [7] , and extracellular neuronal recordings in songbirds [8] , [9] , [10] , [11] , [12] . The more fundamental role of hindbrain pattern generators that directly coordinate and synchronize the activity of vocal musculature, like that of the larynx and avian syrinx, remains relatively unexplored. Prior studies ranging from electromyography to nerve and extracellular neuronal recordings suggest that the hindbrain can determine a vocalization's fine (for example, fundamental frequency) and gross (for example, duration) temporal structure in species as diverse as primates, bats, birds, rodents and frogs [8] , [13] , [14] , [15] , [16] , [17] , [18] , [19] , [20] , [21] , [22] , [23] . Intracellular electrophysiological evidence of how hindbrain neurons determine such traits is sparse, in part, due to a respiratory dependence [24] and concomitant network complexity underlying most tetrapod calling [12] , [13] , [15] , [25] . By contrast, fish provide a unique opportunity to explore hindbrain vocal patterning because the motor network is evolutionarily conserved with other vertebrates, independent of respiration, and directly translated into the natural call attributes of fundamental frequency and duration ( Fig. 1a,b ) [26] , [27] , [28] , [29] . 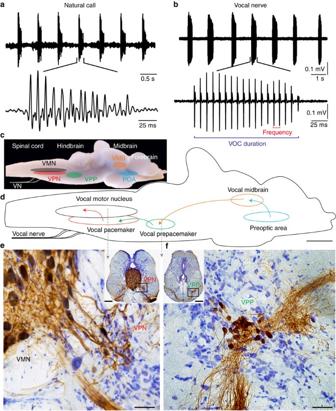Figure 1: Vocal behaviour and neural network of midshipman fish. (a) Oscillograms of natural call series ('grunt train') recorded with hydrophone. (b) Spontaneous neurophysiological responses from vocal nerve with same temporal properties as natural vocalization; lower traces show one call. Duration of VOC response is time between first and last pulse; frequency is the pulse repetition rate. (c) Mapping of vocal motor network superimposed on lateral view of whole brain. (d) Corresponding schematic showing presumed descending control of vocal output, with abbreviations in (c) defined. (e) Transverse section at level indicated indof VMN–VPN circuit transneuronally labelled with biocytin (seemethods); inset shows low magnification view of entire hindbrain at same level. (f) Transverse section at level indicated indof VPP labelled via transneuronal bioctyin transport; inset shows low magnification, bilateral view of VPP. Scale bars: 500 μm in (d) and 25 μm (insets, 200 μm) in (e) and (f). Figure 1: Vocal behaviour and neural network of midshipman fish. ( a ) Oscillograms of natural call series ('grunt train') recorded with hydrophone. ( b ) Spontaneous neurophysiological responses from vocal nerve with same temporal properties as natural vocalization; lower traces show one call. Duration of VOC response is time between first and last pulse; frequency is the pulse repetition rate. ( c ) Mapping of vocal motor network superimposed on lateral view of whole brain. ( d ) Corresponding schematic showing presumed descending control of vocal output, with abbreviations in ( c ) defined. ( e ) Transverse section at level indicated in d of VMN–VPN circuit transneuronally labelled with biocytin (see methods ); inset shows low magnification view of entire hindbrain at same level. ( f ) Transverse section at level indicated in d of VPP labelled via transneuronal bioctyin transport; inset shows low magnification, bilateral view of VPP. Scale bars: 500 μm in ( d ) and 25 μm (insets, 200 μm) in ( e ) and ( f ). Full size image Acoustic communication is widespread among fish, with the best studied being toadfishes, which include midshipman ( Porichthys notatus ), that generate sound by vibrating the swim bladder with a pair of 'drumming' muscles [30] . Midshipman fish are well known for an especially dynamic repertoire of high-frequency vocalizations (fundamental ∼ 100 Hz at 16 °C). Frequency is relatively stable at any one temperature [31] , [32] , with duration among call types varying from ∼ 50 ms to over 1 h (for example, Fig. 1a ) [33] . The temporal properties of these calls is readily recorded from occipital nerve roots ( Fig. 1b ), likely homologues of hypoglossal roots in tetrapods [26] , [29] , that give rise to the nerve innervating the ipsilateral vocal muscle [34] . Retrograde motor neuronal labelling via a single vocal nerve (VN) followed by transneuronal transport delineates a midline pair of motor nuclei and an extensively interconnected network of hindbrain premotor neurons [26] , [35] . The collective output of this premotor-motor network determines the temporal structure of natural calls [28] , [32] , [34] , [36] , [37] . Individual fish vocalizations [30] , [33] (for example, Fig. 1a ), like the notes of avian song [38] and the segments (consonants, vowels) of human speech [39] , [40] , are discrete acoustic elements with no discontinuities along either the time or frequency domain [38] . The current study distinguishes the cellular mechanisms that contribute to the encoding of individual vocal parameters, namely frequency and duration. Using in situ intracellular recordings complemented with structure/function analysis of individual hindbrain neurons in midshipman fish, we show that sustained depolarizations and rhythmic membrane oscillations in separate populations of vocal prepacemaker and downstream pacemaker neurons independently encode the duration and frequency, respectively, of natural vocalizations. Reconstructions of physiologically identified and stained pacemaker neurons show frequency-coding pacemaker axons terminating bilaterally, and nearly exclusively, within the paired vocal motor nuclei. By contrast, duration-coding prepacemaker neurons project throughout the pacemaker-motor neuron circuit as well as to more rostral hindbrain auditory nuclei, including an efferent subgroup innervating the auditory hair cell epithelium of the inner ear. Thus, vocal prepacemaker neurons are the likely source of the known corollary discharge in the audio-vocal network of these fish informing the auditory system about call duration [41] . In summary, our findings propose that premotor segregation of divergent temporal properties allows for an independent and local control of individual vocal parameters in the vertebrate hindbrain. Hindbrain vocal network The vocal motor volley (VOC) is a highly stereotyped series of spike-like waveforms, readily recorded from the vocal occipital nerve roots (VN, Fig. 1b ), that reflects the summed output of the ipsilateral motor nucleus [34] . In vivo intracellular recordings from the hindbrain vocal network ( Fig. 1c–f ), paired with recordings of the rhythmic VOC, identified separate vocal prepacemaker (VPP) and downstream vocal pacemaker nuclei (VPN) encoding call duration and frequency, respectively. The VOC frequency, like natural call frequency (see Introduction), shows little variability ( n =5 fish, 10 VOCs each, mean standard deviation of 3.7% across fish). We electrically evoked (e) VOCs by stimulating midbrain sites (VMB/vocal midbrain, Fig. 1c,d ; trains of 2–10 pulses at 100–300 Hz, presented at intervals of 0.7 s) known to elicit calls in these fish as well as tetrapods [28] , [42] , and compared the observations with spontaneous (s) VOCs. The temporal properties of both sVOCs and eVOCs directly determine the duration and frequency of natural calls and hence serve as reliable proxies for natural vocalizations [32] , [34] , [36] , [37] . We first present anatomical and then electrophysiological results for VPN followed by VPP. Expansive dendritic and axonal arbors of vocal pacemaker neuron Physiologically identified ( n= 63) ( Fig. 2a ; Supplementary Fig. S1a ), neurobiotin-filled ( n= 14) and reconstructed ( n =9) VPN neurons extended along the ventrolateral border of the vocal motor nucleus (VMN) and in nearly all cases exhibited an ovoid-shaped soma together with a bipolar dendritic arbor extending both lateral to and throughout the paired VMN ( Fig. 2b,c ; Supplementary Fig. S1b ). Axons originated from a primary dendrite and then extensively branched, forming prominent synaptic boutons bilaterally throughout the rostral-caudal extent of VMN and VPN ( Fig. 2b–e ; Supplementary Fig. S1b–e ). Two VPN neurons also projected to ipsilateral VPP. In four cases, neighbouring VPN neurons were transneuronally labelled ( n =1.6±0.4 co-labelled neurons), indirectly indicative of gap junctional coupling [35] . VPN's extensive axonal arborizations were thus restricted to the VPP–VPN–VMN network. 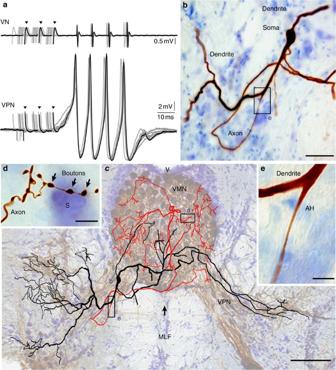Figure 2: Vocal pacemaker neuron morphology. (a) Intracellular vocal pacemaker neuron (VPN, bottom) and corresponding vocal nerve (VN, top) records superimposed with one highlighted (black). All records aligned to first electrically evoked VN waveform. Arrowheads indicate stimulus artefact. (b) Photomicrograph of soma, primary dendrites and axon of neurobiotin-filled VPN neuron. (c) Camera lucida drawing in transverse plane of reconstructed VPN neuron shown in (b). For general context, drawing is superimposed on background image of paired vocal motor nuclei (VMN) (arrow, midline) and VPNs bilaterally filled via transneuronal biocytin transport (brown, cresyl violet counterstain). Axonal (red) and dendritic arbors (black) overlap. (d) Photomicrograph of synaptic boutons in in VMN (S, soma) and (e) of axon hillock (AH) emerging from primary dendrite. Sites shown in (b,d,e) indicated inc. Scale bars represent 50 μm in (b), 100 μm in (c), 10 μm in (d) and 5 μm in (e). MLF, medial longitudinal fasciculi; V, fourth ventricle. Figure 2: Vocal pacemaker neuron morphology. ( a ) Intracellular vocal pacemaker neuron (VPN, bottom) and corresponding vocal nerve (VN, top) records superimposed with one highlighted (black). All records aligned to first electrically evoked VN waveform. Arrowheads indicate stimulus artefact. ( b ) Photomicrograph of soma, primary dendrites and axon of neurobiotin-filled VPN neuron. ( c ) Camera lucida drawing in transverse plane of reconstructed VPN neuron shown in ( b ). For general context, drawing is superimposed on background image of paired vocal motor nuclei (VMN) (arrow, midline) and VPNs bilaterally filled via transneuronal biocytin transport (brown, cresyl violet counterstain). Axonal (red) and dendritic arbors (black) overlap. ( d ) Photomicrograph of synaptic boutons in in VMN (S, soma) and ( e ) of axon hillock (AH) emerging from primary dendrite. Sites shown in ( b , d , e ) indicated in c . Scale bars represent 50 μm in ( b ), 100 μm in ( c ), 10 μm in ( d ) and 5 μm in ( e ). MLF, medial longitudinal fasciculi; V, fourth ventricle. Full size image Oscillatory activity of vocal pacemaker neurons VPNs showed excitatory synaptic inputs at subthreshold stimulation levels for generating eVOCs in the VN ( Fig. 3a ; see Methods for stimulation parameters). As midbrain stimulus amplitude increased, synaptic depolarization gradually grew larger until abruptly ended by a hyperpolarization. A biphasic, oscillatory-like response appeared with successive cycles of synaptic depolarization and hyperpolarization (orange arrows, Fig. 3a ), but without either action potentials or corresponding eVOCs in the VN ( Fig. 3a ). VPN action potentials paired with eVOC potentials appeared with higher midbrain stimulus amplitudes, and at a frequency matching the subthreshold oscillations ( Fig. 3a ). As VPN subthreshold oscillatory activity increased in amplitude and cycle number, superimposed action potentials accompanied each oscillation ( Fig. 3a ). On occasion, a single, smaller amplitude synaptic/action potential depolarization was not correlated with an eVOC potential (black arrows, Fig. 3a ). The smaller amplitude synaptic/action potential sequence, compared with those during the eVOC, likely reflected a reduction in the summed network activity of synchronously firing VPNs (see Discussion ). 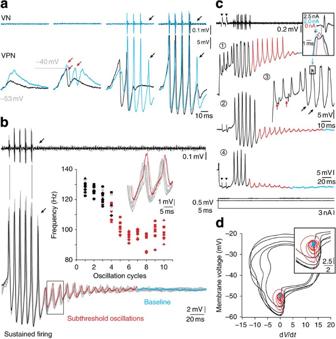Figure 3: Membrane oscillations determine vocal pacemaker neuron firing frequency. (a) Intracellular vocal pacemaker neuron (VPN, bottom) and vocal nerve (VN, top) records colour-coded to show correspondence between VPN and VN records. With increasing depolarizations, membrane oscillations appear that eventually give rise to action potentials. (b) VPN and VN responses superimposed with one response colour–coded to distinguish initial period of sustained action potential firing (black) and subsequent subthreshold oscillations (red) from baseline (blue). Inset: oscillation frequency decreased between the periods of sustained (black) and subthreshold (red) activity; subthreshold oscillations from box. (c) Neuron in (b) during current injection. Trace 1 shows subthreshold oscillations of trace 2 (the response during no current injection) replaced by action potentials during depolarizing current injection. Trace 3, taken from the beginning of trace 1, shows small (red arrows) and prominent (black arrows) after-hyperpolarizations prior to and after first VN waveform, respectively. Depolarizing current injection also leads to changes in action potential shape. The box adjacent to trace 1 shows three expanded records of same neuron at different levels of depolarizing current injection, colour-coded to show different spike shapes aligned to corresponding eVOC spike (hatched line); 0.0 nA red record from trace 2 and 2.0 nA blue record from action potential in trace 3 as indicated by blue arrow. Trace 4 shows decreased action potential and subthreshold oscillation amplitudes during hyperpolarizing current injection, although the oscillations never completely disappear. Arrowheads indicate stimulus artefact. (d) Phase plane plot of VPN activity in neuron in (b). Action potential firing is stable during the eVOC (black spirals), whereas subthreshold oscillations dampen in amplitude (red spirals) as the response returns to baseline (blue). Figure 3: Membrane oscillations determine vocal pacemaker neuron firing frequency. ( a ) Intracellular vocal pacemaker neuron (VPN, bottom) and vocal nerve (VN, top) records colour-coded to show correspondence between VPN and VN records. With increasing depolarizations, membrane oscillations appear that eventually give rise to action potentials. ( b ) VPN and VN responses superimposed with one response colour–coded to distinguish initial period of sustained action potential firing (black) and subsequent subthreshold oscillations (red) from baseline (blue). Inset: oscillation frequency decreased between the periods of sustained (black) and subthreshold (red) activity; subthreshold oscillations from box. ( c ) Neuron in ( b ) during current injection. Trace 1 shows subthreshold oscillations of trace 2 (the response during no current injection) replaced by action potentials during depolarizing current injection. Trace 3, taken from the beginning of trace 1, shows small (red arrows) and prominent (black arrows) after-hyperpolarizations prior to and after first VN waveform, respectively. Depolarizing current injection also leads to changes in action potential shape. The box adjacent to trace 1 shows three expanded records of same neuron at different levels of depolarizing current injection, colour-coded to show different spike shapes aligned to corresponding eVOC spike (hatched line); 0.0 nA red record from trace 2 and 2.0 nA blue record from action potential in trace 3 as indicated by blue arrow. Trace 4 shows decreased action potential and subthreshold oscillation amplitudes during hyperpolarizing current injection, although the oscillations never completely disappear. Arrowheads indicate stimulus artefact. ( d ) Phase plane plot of VPN activity in neuron in ( b ). Action potential firing is stable during the eVOC (black spirals), whereas subthreshold oscillations dampen in amplitude (red spirals) as the response returns to baseline (blue). Full size image In 9 of 14 somato-dendritic recordings, subthreshold membrane oscillations persisted after an initial period of uninterrupted (sustained) action potential firing matched 1:1 with eVOC spikes ( Fig. 3b ). Subthreshold oscillations were not observed in either VPN axonal recordings ( n= 10) or within any motor neuronal compartment recordings ( n =28; see methods/data analysis for recording site distinction). Subthreshold oscillation amplitudes did not exceed a certain level of membrane depolarization, strongly indicating a voltage dependency of the oscillations ( Fig. 3b inset). Oscillation frequency gradually decreased during the subthreshold responses ( Fig. 3b inset) and was significantly different between the periods of sustained action potential firing and subthreshold activity (last 4 cycles of sustained: 123.3±2.5 Hz; first 4 cycles of subthreshold: 98.48±1.3 Hz; paired t -test: P <0.001). Positive and negative current clamp manipulation of the resting potential during eVOCs had no significant effect on the firing frequency of the sustained action potential response (Mann-Whitney U test: positive current, P =0.59; Mann-Whitney U test: negative current, P =0.52). However, with positive current injection, subthreshold oscillations were replaced by action potentials at the subthreshold frequency (Mann-Whitney U test, P =0.24), but without concurrent eVOC spikes ( Fig. 3c , trace 1; trace 2 shows baseline activity). Compared with action potentials induced by positive current injection alone ( Fig. 3c ; red arrows in trace 3, expanded from beginning of trace 1), the synaptic/action potential sequence showed a much larger after-hyperpolarization during eVOCs ( Fig. 3c , black arrows in trace 3). Although membrane hyperpolarization significantly decreased subthreshold frequency compared with baseline (Mann-Whitney U test: 94.7 Hz±3.4 Hz, P <0.01), the oscillations never completely disappeared ( Fig. 3c , trace 4). Positive current injection during eVOCs also resulted in small double peaks in VPN action potentials ( Fig. 3c , blue arrow in trace 3). The distance between the two peaks increased in proportion to higher currents, but the second peak was phase-locked to the eVOC spike ( Fig. 3c box). The latency shift in peak 1 reflected the earlier onset of the recorded neuron's electrical response during the network oscillatory activity (peak 2) (also see Discussion ). To test whether single neurons could intrinsically generate an oscillatory pattern like the one during eVOCs, we elicited action potentials during EPSPs in VPN neurons ( n =4). None of the VPN neurons showed either sustained oscillatory firing or subthreshold oscillations after action potentials were elicited, further suggesting the role of a VPN network in generating vocal responses ( Supplementary Fig. S1f,g ). The frequency of action potential firing, subthreshold oscillations and eVOCs was independent of midbrain stimulation frequency (ANOVAs; P values >0.26). A phase-plane plot revealed the stability of VPN firing throughout the eVOC (black spirals; Fig. 3d ), but not after the eVOC during subthreshold oscillations when the activity spiralled in (red spirals; Fig. 3d ) towards the resting potential (blue; Fig. 3d ). More significantly, VPN sustained (that is, continuous firing) and subthreshold oscillatory responses did not differ between more naturalistic sVOCs and eVOCs ( Figs 3b,d and 4a ). 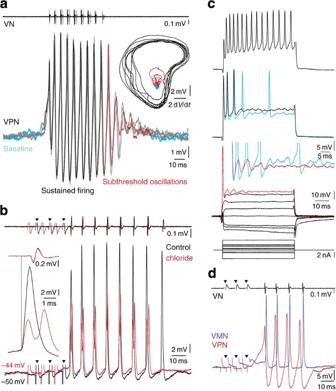Figure 4: Spontaneous vocal pacemaker neuron responses and effects of chloride injections. (a) Spontaneous vocal pacemaker neuron (VPN, bottom) and corresponding vocal nerve (VN, top) responses are superimposed with one response colour–coded to distinguish the initial period of sustained firing of action potentials (black) and subsequent subthreshold oscillations (red) from baseline (blue). Inset shows phase plane plot of neuronal activity (onset activity not included). Action potential firing is highly stable during sVOC (black spirals), whereas subsequent subthreshold oscillations gradually dampen in amplitude (red spirals) as the response returns to baseline (blue). (b) VPN (bottom) and VN (top) activity before (control, black) and after chloride (red) injection during electrically evoked responses. Action potentials compared on slower time scale in inset. (c) Responses following increasing levels of intracellular current injection (bottom to top, for example, red: 1.52 nA, blue: 1.78 nA). Amplified action potentials (truncated) in inset above first set of records are colour-coded for clarity. With increasing membrane depolarization (from bottom to top traces), subthreshold oscillations not present in resting membrane potential (bottom trace) become apparent and were accompanied by action potentials (for example, red and blue traces), eventually resulting in tonic firing (top black trace). (d) Alignment of first VN waveform (top) and intracellular records (bottom) from single vocal motor (VMN, blue) and VPN (red) neurons. Arrowheads in (b,d) indicate stimulus artefact. Figure 4: Spontaneous vocal pacemaker neuron responses and effects of chloride injections. ( a ) Spontaneous vocal pacemaker neuron (VPN, bottom) and corresponding vocal nerve (VN, top) responses are superimposed with one response colour–coded to distinguish the initial period of sustained firing of action potentials (black) and subsequent subthreshold oscillations (red) from baseline (blue). Inset shows phase plane plot of neuronal activity (onset activity not included). Action potential firing is highly stable during sVOC (black spirals), whereas subsequent subthreshold oscillations gradually dampen in amplitude (red spirals) as the response returns to baseline (blue). ( b ) VPN (bottom) and VN (top) activity before (control, black) and after chloride (red) injection during electrically evoked responses. Action potentials compared on slower time scale in inset. ( c ) Responses following increasing levels of intracellular current injection (bottom to top, for example, red: 1.52 nA, blue: 1.78 nA). Amplified action potentials (truncated) in inset above first set of records are colour-coded for clarity. With increasing membrane depolarization (from bottom to top traces), subthreshold oscillations not present in resting membrane potential (bottom trace) become apparent and were accompanied by action potentials (for example, red and blue traces), eventually resulting in tonic firing (top black trace). ( d ) Alignment of first VN waveform (top) and intracellular records (bottom) from single vocal motor (VMN, blue) and VPN (red) neurons. Arrowheads in ( b , d ) indicate stimulus artefact. Full size image Frequency-coding vocal pacemaker neurons Given the role of inhibition in coupling the activity of neuronal populations [43] , [44] , [45] , we tested the hypothesis that the hyperpolarizing membrane activity seen during VPN oscillations might arise from network inhibitory action. At subthreshold stimulation levels for generating eVOCs, VPN recordings ( n =4) did not show any change in membrane potential after chloride (Cl − ) injection in the somatodendritic compartment via 2 M KCl-filled electrodes. Neither the action potentials during eVOCs nor the following subthreshold oscillations differed from those in non-chloride injected neurons. A Cl − effect could, however, be detected in axonal recordings. Following Cl − injection, VPN axonal recordings ( n =6) ( Fig. 4b ) exhibited two distinct depolarizations. Onset of the first component coincided with the shortest latency depolarization that could be either the synaptic component (that is, the coupled network) or the initial segment action potential. The change in action potential shape also served as a control for successful loading of Cl − into VPNs. Independent of either the site or extent of Cl − injected, VPN firing frequency did not change ( Fig. 4b ), hence we concluded that inhibitory inputs to VPN neurons were not the origin of oscillatory VPN activity. We next investigated the response properties of VPN neurons ( n= 4) to current steps with varying amplitudes ( Fig. 4c ). With increasing membrane depolarization, subthreshold oscillations not present at resting membrane potentials became apparent and were eventually accompanied by action potentials. Further increases in current amplitude resulted in tonic action potential firing at frequencies >300 Hz. The time course of VPN action potentials always matched that of vocal motor neurons and the eVOC/sVOC. Temporal alignment of sequentially recorded VPN and VMN action potentials showed VPNs ( n =10) firing 1.25±0.3 ms prior to VMN neurons and eVOCs ( Fig. 4d ). Despite their similarity in firing frequency, VMN neurons, unlike VPNs, did not display any subthreshold oscillatory activity or membrane oscillations during current injection (B. Chagnaud, M. Zee, R. Baker, A. Bass, unpublished observation). The extensive innervation of VMNs by single VPNs ( Fig. 2d ; Supplementary Fig. S1b ), together with the evidence for VPN activity as the oscillatory potential complex, supports VPN's role in setting motor neuron firing frequency and, in turn, natural call frequency. Vocal prepacemaker neurons project within and outside the vocal system Physiologically identified ( n =54), neurobiotin-filled ( n =16) and reconstructed ( n =9) VPP neurons had 2–5 major dendritic branches that divided into smaller branches with increasing distance from the soma ( Fig. 5a–c ). Ventromedial branches extended across the midline ( Fig. 5c ), with varicose-like expansions along smaller branchlets near the ventral midline. Axons arose from either a primary dendrite or the soma ( Fig. 5d ). Extensive trans-neuronal labelling of adjacent VPP neurons ( n =16.1±9) ( Fig. 5e ) accompanied most single neuron injections ( n =7), consistent with a hypothesized widespread gap junction coupling [35] . 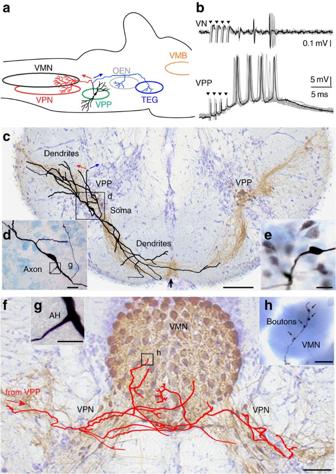Figure 5: Vocal prepacemaker neuron morphology. (a) Line drawing of sagittal view showing location of reconstructed vocal prepacemaker (VPP) neuron soma and dendrites (black), and axon with rostral (blue) and caudal (red) branches. OEN (grey); TEG (blue); VMB (orange); VMN (black); VPN (red); VPP (green). (b) Intracellular records (bottom) of reconstructed neuron with corresponding vocal nerve activity (VN, top); superimposed records with one highlighted (black). Arrowheads indicate stimulus artefact. (c) Camera lucida drawing in transverse plane of reconstructed VPP neuron. For ease of visibility, drawing superimposed on background image of transneuronally labelled VPP nuclei (brown, cresyl violet counterstain). Dendritic arbor (black) extends across midline (vertical black arrow). Colour-coded arrows correspond to those inashowing axon bifurcation into rostral and caudal branches. (d) Photomicrograph of axon arising from primary dendrite (see box inc) and (e) of neighbouring VPP neurons transneuronally labelled after single VPP neuron injection. (f) Reconstruction of VPP caudal axonal arbor superimposed on image of transneuronally labelled vocal motor (VMN) and pacemaker (VPN) neurons. (g) Photomicrograph of axon hillock (AH, see box ind) and (h) of terminal boutons over a cresyl-violet stained soma in VMN (see box inf). Scale bars represent 100 μm in (c,f), 25 μm in (d,e), 10 μm in (g,h). Figure 5: Vocal prepacemaker neuron morphology. ( a ) Line drawing of sagittal view showing location of reconstructed vocal prepacemaker (VPP) neuron soma and dendrites (black), and axon with rostral (blue) and caudal (red) branches. OEN (grey); TEG (blue); VMB (orange); VMN (black); VPN (red); VPP (green). ( b ) Intracellular records (bottom) of reconstructed neuron with corresponding vocal nerve activity (VN, top); superimposed records with one highlighted (black). Arrowheads indicate stimulus artefact. ( c ) Camera lucida drawing in transverse plane of reconstructed VPP neuron. For ease of visibility, drawing superimposed on background image of transneuronally labelled VPP nuclei (brown, cresyl violet counterstain). Dendritic arbor (black) extends across midline (vertical black arrow). Colour-coded arrows correspond to those in a showing axon bifurcation into rostral and caudal branches. ( d ) Photomicrograph of axon arising from primary dendrite (see box in c ) and ( e ) of neighbouring VPP neurons transneuronally labelled after single VPP neuron injection. ( f ) Reconstruction of VPP caudal axonal arbor superimposed on image of transneuronally labelled vocal motor (VMN) and pacemaker (VPN) neurons. ( g ) Photomicrograph of axon hillock (AH, see box in d ) and ( h ) of terminal boutons over a cresyl-violet stained soma in VMN (see box in f ). Scale bars represent 100 μm in ( c , f ), 25 μm in ( d , e ), 10 μm in ( g , h ). Full size image VPP axons often bifurcated at VPP levels into rostral and caudal branches ( Fig. 5a ). In most cases ( n =7), the caudal branch targeted VPN-VMN bilaterally ( Fig. 5f ) with a subset ( n =2) projecting to both VPN-VMN and the contralateral VPP ( Supplementary Fig. S2a–c ). Rostral hindbrain terminals overlapped the dense primary dendritic region of the central (octavolateralis) efferent nucleus (OEN) that directly innervates the inner ear and lateral line organs ( Fig. 5a ). Terminals were also found directly over a tegmental nucleus (TEG, Fig. 5a , Supplementary Fig. S2a ) that is a ventral extension of an VIIIth nerve-recipient auditory nucleus [35] , [46] . The axons of two VPP neurons extended to midbrain levels ( Supplementary Fig. S2a–f ). Two other VPP axons did not project to VPN-VMN, with one extending at least 300 μm into the spinal cord ( Supplementary Fig. S3a–d ) and the other exclusively to the facial motor nucleus. Thus, unlike VPNs, VPP neurons had extensive projections outside the VPP-VPN-VMN network, most prominently to hindbrain auditory regions. Duration coding by vocal prepacemaker neurons Intracellular records were obtained from 54 VPP neurons during the production of sVOCs and eVOCs in the vocal nerve (VN, Fig. 6 ). Unlike VPN neurons, VPP neurons ( n =6) did not show membrane oscillations in response to current steps. Instead, they only responded with tonic firing that increased in frequency with increasing current ( Fig. 6a ). To investigate the underlying mechanisms of VPP activity, the membrane potential was hyperpolarized below action potential threshold. VPP neurons generated a sustained depolarization that began prior to the first sVOC pulse and outlasted the entire call ( Fig. 6b ). The duration of the depolarization (half-width of the response) showed a strong linear relationship (linear regression: y=0.9*x+30.2; R 2 =0.983, P <0.001) with corresponding sVOC duration (interval between first and last sVOC waveform, Fig. 6c ). Sustained depolarizations were not apparent upon intracellular current injection ( Fig. 6a ). 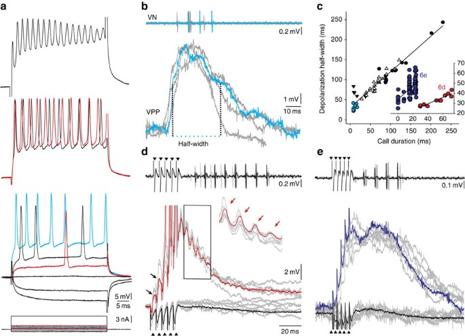Figure 6: Temporal coding of call duration by vocal prepacemaker neurons. (a) Vocal prepacemaker (VPP) neuron responses (colour-coded for clarity) following increasing levels of intracellular current injection (bottom to top, for example, lower red: 0.34 nA, blue: 0.78 nA). VPP neurons fired an increasing number of action potentials with increasing membrane depolarization in response to current steps, but did not show membrane oscillations (bottom three red, black and blue traces). VPP neurons eventually responded with tonic firing that increased in frequency with increasing current (top three red and black traces). (b) Spontaneous vocal nerve (VN, top) and corresponding intracellular VPP (bottom) activity superimposed with one trace highlighted (blue). Half-width of sustained depolarization indicated with dotted lines. (c) Linear regression showing relationship between duration of spontaneous VN response and half width of sustained depolarization. Each symbol represents a different neuron (n=4) with multiple trials per neuron; light blue-filled symbols represent neuron shown inb. Similar depiction in inset for electrically evoked neuronal responses (d, red ande, dark blue). (d) Midbrain-evoked VPP (bottom) and corresponding VN (top) activity superimposed with one record highlighted in red. Neuron shows peak activity at beginning of VN response and EPSPs (black arrows). Neuron displayed oscillations (box) magnified in inset (superimposed records with one highlighted in red trace with arrows). The VPP response was more prolonged, but less tightly correlated (inset inc) with the duration of VN activity than the neuron ine. (e) Midbrain-evoked VPP (bottom) and corresponding VN (top) activity superimposed with one record highlighted in blue. Arrowheads ind,eindicate stimulus artefact. Figure 6: Temporal coding of call duration by vocal prepacemaker neurons. ( a ) Vocal prepacemaker (VPP) neuron responses (colour-coded for clarity) following increasing levels of intracellular current injection (bottom to top, for example, lower red: 0.34 nA, blue: 0.78 nA). VPP neurons fired an increasing number of action potentials with increasing membrane depolarization in response to current steps, but did not show membrane oscillations (bottom three red, black and blue traces). VPP neurons eventually responded with tonic firing that increased in frequency with increasing current (top three red and black traces). ( b ) Spontaneous vocal nerve (VN, top) and corresponding intracellular VPP (bottom) activity superimposed with one trace highlighted (blue). Half-width of sustained depolarization indicated with dotted lines. ( c ) Linear regression showing relationship between duration of spontaneous VN response and half width of sustained depolarization. Each symbol represents a different neuron ( n =4) with multiple trials per neuron; light blue-filled symbols represent neuron shown in b . Similar depiction in inset for electrically evoked neuronal responses ( d , red and e , dark blue). ( d ) Midbrain-evoked VPP (bottom) and corresponding VN (top) activity superimposed with one record highlighted in red. Neuron shows peak activity at beginning of VN response and EPSPs (black arrows). Neuron displayed oscillations (box) magnified in inset (superimposed records with one highlighted in red trace with arrows). The VPP response was more prolonged, but less tightly correlated (inset in c ) with the duration of VN activity than the neuron in e . ( e ) Midbrain-evoked VPP (bottom) and corresponding VN (top) activity superimposed with one record highlighted in blue. Arrowheads in d , e indicate stimulus artefact. Full size image In response to midbrain electrical stimulation, VPP neurons exhibited an EPSP immediately following each stimulus pulse, suggesting a monosynaptic midbrain input (black arrows, Fig. 6d ). EPSPs summated with each subsequent stimulus until either reaching a saturation level or an action potential threshold ( Fig. 6d ). Following midbrain stimulation, the membrane potential did not immediately return to baseline. Rather, VPP neurons exhibited a sustained depolarization with a more ( Fig. 6e ) or less ( Fig. 6d ) uniform, prolonged duration similar to responses during sVOCs ( Fig. 6b ). The membrane potential did not return to baseline until after call cessation and, as with sVOCs, was significantly correlated with call duration ( Fig. 6c inset; linear regressions were y=0.70*x+33.6, R 2 =0.86, P <0.001 for data corresponding to Fig. 6d and y=0.29*x+18.6, R 2 =0.37, P <0.001 for data corresponding to 6e). A subset of VPP neurons ( n =3) also generated prominent oscillations (red arrows in inset of Fig. 6d ), but at a frequency different from the midbrain stimulus, eVOC or pacemaker (VPN) neurons. Manipulation of vocal prepacemaker affects call duration VPP's role in setting call duration was further tested by injections of lidocaine that selectively inactivates voltage-gated sodium channels essential for action potential propagation. On average, the eVOC was completely abolished and duration plummeted to zero within 5 min after bilateral VPP injections ( n =8) ( Fig. 7a ; blue traces in Fig. 7b ). Vocal activity gradually returned to baseline levels by 40 min post-injection ( Fig. 7a,b ). Lidocaine had no effect on call frequency ( Fig. 7b ) (Wilcoxon test: Z=−1.84, P =0.066). Bilateral control injections (vehicle/0.1 M PB alone, n =9; black traces in Fig. 7b ) showed no significant effect on either duration or frequency (Wilcoxon test: duration, Z=−2.17, P =0.940; Wilcoxon test: frequency, Z=−1.33, P =0.182). In three cases with a unilateral VPP lidocaine injection, a reversible decrease in call duration also occurred with no change in frequency ( Fig. 7b , red traces). Unlike bilateral injections, the call did not disappear ( Fig. 7b ). Labelling of injection sites with fluorescent dextran amine revealed that all injections were in VPP (vehicle only, n =2; vehicle plus lidocaine, n =5). 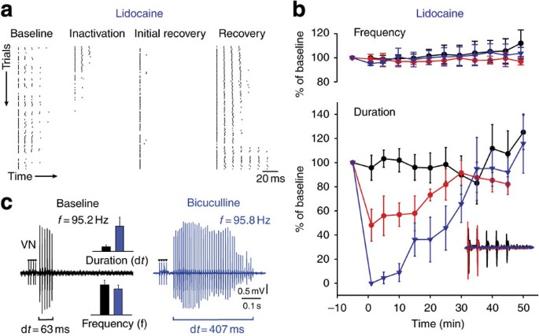Figure 7: Pharmacological activation and inactivation of vocal prepacemaker neurons. (a) Raster plots show 100 consecutive trials of vocal nerve (VN) activity (each point represents a single VN potential) at baseline (t=−5 min) and then three post-injection time points after bilateral lidocaine injection into vocal prepacemaker nucleus: inactivation (3 min), initial recovery (20 min) and full recovery (40 min). (b) Summary of changes (normalized to baseline levels; mean±standard error of the mean) in VN frequency and duration following bilateral (n=8, blue) and unilateral (n=3, red) lidocaine injections, and after-control (0.1 M phosphate buffer) injections (n=11, black). Inset in duration summary shows representative VN responses. (c) Midbrain evoked vocal nerve activity at baseline (black) and after bilateral bicuculline injection into VPP (blue). Changes in duration and frequency between baseline and 5 min after injection shown in bar graph insets. Arrowheads indicate stimulus artefact. Figure 7: Pharmacological activation and inactivation of vocal prepacemaker neurons. ( a ) Raster plots show 100 consecutive trials of vocal nerve (VN) activity (each point represents a single VN potential) at baseline ( t =−5 min) and then three post-injection time points after bilateral lidocaine injection into vocal prepacemaker nucleus: inactivation (3 min), initial recovery (20 min) and full recovery (40 min). ( b ) Summary of changes (normalized to baseline levels; mean±standard error of the mean) in VN frequency and duration following bilateral ( n =8, blue) and unilateral ( n =3, red) lidocaine injections, and after-control (0.1 M phosphate buffer) injections ( n =11, black). Inset in duration summary shows representative VN responses. ( c ) Midbrain evoked vocal nerve activity at baseline (black) and after bilateral bicuculline injection into VPP (blue). Changes in duration and frequency between baseline and 5 min after injection shown in bar graph insets. Arrowheads indicate stimulus artefact. Full size image Given the presence of GABAergic neurons within VPP (M. Zee, A. Bass, unpublished observation), we tested the role of inhibition in determining call duration by injecting bicuculline, a competitive GABA A receptor antagonist, into VPP. Bilateral injections ( n =4) of bicuculline resulted in a significant increase of eVOC duration ( Fig. 7c ): baseline (black trace and black in duration bar graph): 39.9±16.8 ms; post-injection (blue trace and blue in bar graph): 245.9±69 ms; t -test: P =0.003), indicative of an inhibitory action on VPP. There was no significant effect on frequency ( t -test: P =0.940) ( Fig. 7c , frequency bar graph). We demonstrate that timing signals for both fine (frequency) and gross (duration) temporal structure, basic features shared by elemental vocal units among vertebrates [33] , [38] , [39] , [40] , are coded by separate hindbrain premotor populations ( Fig. 8 ). The hindbrain-spinal region surgically isolated in situ that includes the VPP–VPN–VMN network can generate a vocal motor output completely predicting the temporal properties of natural calls [36] , [37] . The inherent rhythmicity and synchronicity of this vocal compartment depend, in part, on extensive coupling between all component nuclei, eventually leading to simultaneous contraction of the vocal muscles and generation of natural calls at frequencies within the gamma-ultrafast range. Despite the pervasive interconnectivity within this network that might imply multifunctional properties for its component neurons, separate premotor nuclei exhibit distinct physiological profiles. While this compartmentalization may be a general feature of hindbrain premotor organization in either fish [47] or vertebrates in general, it is consistent with a wide range of extracellular recording studies in amphibians, birds and mammals (including primates) that show neural activity correlated with either vocalization duration or frequency (see Introduction). 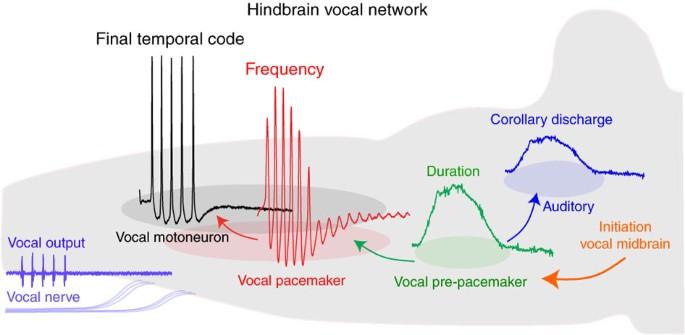Figure 8: Summary of connectivity of vocal hindbrain network and temporal code. Shown are representative intracellular records from vocal prepacemaker, pacemaker and motor neurons, and vocal nerve activity superimposed on background sagittal image of caudal hindbrain. Hindbrain vocal activity is initiated by descending input from vocal midbrain neurons. The vocal prepacemaker nucleus also innervates auditory nuclei, providing a corollary discharge that informs the auditory system about the temporal attributes of natural vocalizations. The results suggest that premotor compartmentalization of neurons coding distinct acoustic attributes is a fundamental trait of hindbrain vocal pattern generators among all vocal vertebrates, including birds and mammals. Figure 8: Summary of connectivity of vocal hindbrain network and temporal code. Shown are representative intracellular records from vocal prepacemaker, pacemaker and motor neurons, and vocal nerve activity superimposed on background sagittal image of caudal hindbrain. Hindbrain vocal activity is initiated by descending input from vocal midbrain neurons. The vocal prepacemaker nucleus also innervates auditory nuclei, providing a corollary discharge that informs the auditory system about the temporal attributes of natural vocalizations. The results suggest that premotor compartmentalization of neurons coding distinct acoustic attributes is a fundamental trait of hindbrain vocal pattern generators among all vocal vertebrates, including birds and mammals. Full size image Several lines of evidence indicate that VPN neurons encode motor neuronal (VMN) firing rate, hence natural call frequency. VPN neurons had expansive, bilateral axonal arborizations throughout VMN. During spontaneous and midbrain-evoked vocal activity (sVOC/eVOC), VPN neurons displayed oscillatory activity directly matching VMN and VOC frequency, with each cycle of VPN sustained firing preceding a VMN action potential. Whereas the membrane oscillations of individual VPN neurons increased in number and frequency with increasing current injection, a prerequisite for oscillations [48] , several observations suggest that VPN oscillations during VOCs, and hence natural vocalization, arise from network activity. During current injection alone, there was a distinct absence of prominent after-hyperpolarizations and sustained/subthreshold potentials at a fixed frequency as observed during VOCs. Although current injection alone could drive VPN oscillatory frequency to far exceed VOC frequency, firing frequency was unchanged during VOCs when either depolarizing or hyperpolarizing current was injected. Thus, despite the intrinsic ability of VPN neurons to oscillate over a wide range of frequencies, network properties apparently constrain oscillation frequency. Positive current injection during VOCs led to VPN action potentials with double peaks that represented the activity of the recorded VPN neuron itself and the network activity of electrotonically coupled VPN neurons (peaks 1 and 2, respectively, Fig. 3c box). However, there was no significant shift in action potential frequency because of network predominance in setting frequency. Lastly, eliciting an action potential during subthreshold activity ( Supplementary Fig. S1f,g ) did not lead to oscillatory activity. The high degree of synchronous activity of the VPN network likely depends, in part, on gap junction coupling as demonstrated for the inferior olive [44] , [45] . Labelling of neighbouring VPN neurons following single VPN neuron injections, along with extensive transneuronal transport throughout VPN and VMN following biocytin application to one vocal nerve [35] , suggests extensive gap junctional coupling in VPN. Amplitude fluctuations of the membrane potential at the VOC frequency (black arrows, Fig. 3a ) indicate variation in summed network activity that could be, in part, mediated by electrotonic coupling of VPNs. The presence of electrotonic coupling, known to be involved in the generation and maintenance of synchronized firing [49] , could thus be an important factor determining VPN network activity. We conclude that VPN essentially functions as a synchronizing conditional oscillator, well adapted for excitatory drive to the 'superfast' vocal muscles shared by fish and other vertebrates [50] . In particular, oscillatory activity occurs on a timescale comparable to rapid temporal modulations in tetrapod vocalizations [13] , [15] , [51] , [52] . All of the evidence presented indicates that VPP is the critical node in the vocal hindbrain network determining call duration. The duration of VPP sustained depolarizations showed a strong linear relationship with call duration. Somatic current injection did not lead to sustained depolarizations indicating, together with the exponential decay during the repolarizing phase of VPP activity ( Fig. 6 ), that a metabotropic mechanism [53] likely contributes to the generation of sustained depolarizations. Injections into VPP of lidocaine and the GABA A receptor antagonist bicuculline induced a rapid (within 5 min) decrease and increase in call duration, respectively. Whereas we did not directly demonstrate the effect of either bicuculline or lidocaine on single VPP neurons, the rapid change in VOC duration after pharmacological application indicated a local effect. VPP's abundant expression of androgen receptor messenger RNA [54] and dense peptidergic input [55] , together with rapid androgen and neuropeptide dependent modulation of call duration [36] , [37] , [56] , is also indicative of VPP's essential role in setting this temporal parameter. Thus, dynamic modulation of the duration of VPP's sustained depolarizations, and in turn natural calls, is likely achieved via direct GABAergic and hormonal control. VPP is a critical node linking the vocal and auditory systems. Unlike VPN connectivity that is confined to the hindbrain vocal motor network, VPP uniquely also projects to auditory nuclei. This includes an efferent subgroup that innervates the inner ear (OEN, Fig. 5a ) and mediates the known vocal corollary discharge [41] , along with an eighth nerve-recipient hindbrain tegmental nucleus (TEG, Fig. 5a ) acting as a prominent audio-vocal interface in the ascending auditory system [46] . Whereas the tegmental pathway may serve as a corollary discharge to filter reafferent signals during auditory processing [57] , the projection to the inner ear's efferent nucleus directly modulates peripheral auditory sensitivity to self-generated sounds and would therefore reduce reafferent stimulation caused by one's own vocalization [41] . This finding provides a novel preparation for investigating how central efferent input to the inner ear, a pathway shared among all vertebrates [58] , can actively modify peripheral auditory function including the cochlea [59] . We show premotor segregation of neurons with intrinsic and network properties adapted for patterning fine (frequency) and gross (duration) temporal structure in a highly conserved, hindbrain vocal network, with proposed VPN counterparts [26] in premotor avian (retroambigualis/parambigualis) [8] , [12] , [25] and mammalian, including primate, (peri-ambigual reticular formation/dorsal reticular) [14] , [16] , [60] nuclei. The parsing of frequency- and duration-coding neurons into separate populations provides a basis for both the independent control of discrete vocal parameters and their separate influences on the auditory system mediated by corollary discharge pathways ( Fig. 8 ). Whereas the songs of birds and speech of humans are more complex, the final premotor control of individual vocal parameters may depend on multiple hindbrain populations, each with a predominant temporal coding task. This organizational pattern would complement upstream forebrain vocal nuclei with distinct coding functions [8] , [9] , [10] , [11] . Animals This study included 81 midshipman fish (standard length range: 4.5–18.7 cm; mean: 12.89±2.88 cm). Midshipman have two male morphs [31] . Only type I males that acoustically court females were used in this study [31] . Animals were collected either from intertidal nest sites or by offshore trawls in northern California. Animals were housed in isolation with a light–dark cycle of 14h: 10 h at 16–17 °C. All animal procedures were approved by the Cornell University and the Marine Biological Laboratory Institutional Animal Care and Use Committees. Surgery Surgical procedures followed previously described methods [34] , [42] . Briefly, fish were first anaesthetized by immersion in 0.025% ethyl p-amino benzoate (Sigma) dissolved in artificial seawater. Bupivacaine (0.25%; Abbot Laboratories) with 0.01 mg ml −1 epinephrine (International Medication Systems) was injected near the wound site for long-term anaesthesia. A dorsal craniotomy exposed the brain and rostral spinal cord, and the paired ventral occipital nerve roots that innervate the vocal muscles [34] . Animals were given intramuscular injections of pancuronium bromide (0.5 mg per kg body weight; Astra Pharmaceutical Products) for immobilization and then transferred to the experimental tank that rested on a vibration isolation table (TMC). A tube inside the fish's mouth provided recirculated chilled (16±3 °C) salt water across the gills. Stimulation Vocalizations were evoked by current pulses delivered to vocal midbrain areas via insulated tungsten electrodes (5 MΩ impedance; A-M Systems) [27] , [34] , [42] . Current pulses were delivered via a constant current source (model 305-B, World Precision Instruments). A stimulus generator (A310 Accupulser, World Precision Instruments) was used to generate TTL pulses with a standard search stimulus of 5 pulses at 200 Hz. Each pulse train equalled one stimulus delivery with interstimulus intervals of 0.7 s. During recordings, interpulse intervals (range: 100–300 Hz) and total pulse number (2–10) varied. The evoked vocal motor volley (eVOC) was monitored with an extracellular electrode (75 μm diameter Teflon-coated silver wire with an exposed ball tip, 125–200 μm in diameter) placed on one of the vocal occipital nerve roots [34] . The vocal nerves exiting from both sides of the hindbrain fire in phase so that the recordings from one side reflect the bilateral pattern of activation of the paired vocal muscles [34] . Nerve recordings were amplified 1,000-fold and band-pass filtered (300–5 kHz) with a differential AC amplifier (Model 1700, A-M Systems). Spontaneous (s) VOCs were also recorded. Neurophysiological recordings Intracellular glass micropipettes (A-M systems) were pulled on a horizontal puller (P97, Sutter Instruments) and filled with 5% neurobiotin (Vector Laboratories) in 0.5 M potassium acetate (resistance: 35–60 MΩ). Neuronal signals were amplified 100-fold (Biomedical Engineering) and digitized at a rate of 20 kHz (Digidata 1322A, Axon Instruments/Molecular Devices) using the software pclamp 9 (Axon Instruments). An external clock (Biomedical Engineering) sending TTL pulses was used to synchronize stimulus delivery and data acquisition. Electrode resistance was monitored while searching for neurons by a current step applied to the recording electrode. To decrease the electrical artefact produced by the midbrain current stimulation, grounded aluminium foil was used to shield the recording electrodes from the midbrain stimulation electrode. Single cell anatomy For intracellular staining of recorded neurons, positive current (range: 3–7 nA) with a duty cycle of 50% at 2–4 Hz was passed through a neurobiotin-filled recording electrode for 3–10 min (see above). Fish were deeply anaesthetized (0.025% benzocaine) 4–6 h after neurobiotin injection, followed by transcardial perfusion with cold, teleost Ringer solution and a solution of 3.5% paraformaldehyde/0.5% glutaraldehyde in 0.1 M phosphate buffer (PB). Brains were postfixed (2–12 h) and then transferred to 0.1 M PB (pH 7.2) for storage. Brains were cryoprotected in 30% sucrose-PB (overnight), embedded in 15% gelatin and sectioned (100 or 120 μm thick) in the transverse plane on a sliding microtome. Floating sections were reacted with an ABC kit (Vector Laboratories), mounted on gelatin-coated slides, and counterstained with cresyl violet. Neurobiotin-filled neurons were reconstructed at a magnification of ×400 using a camera lucida attachment (Leitz Orthoplan microscope). Drawings were scanned and images further processed with the software Photoshop 7.0 and Corel draw. Photographs of selected sections were taken with a digital camera (Spotflex model 15.2, Diagnostic Instruments; attached to Nikon Eclipse E800 microscope) and were postprocessed with Photoshop 7.0 for contrast and brightness enhancement. Photographs of sections were taken at different image depths and image stacks were merged for presentation using Photoshop. Reconstructed neurons were superimposed on images of transneuronally labelled, biocytin-filled VPP–VPN–VMN circuit following labelling of a single vocal nerve [35] . Data analysis Putative microelectrode recording sites in individual neurons were determined using rise time and action potential half-width. Axonal recordings exhibited abruptly arising action potentials with half-widths less of 0.72±0.11 ms. In contrast, somatic and dendritic recordings showed broader action potentials with spike half-width of 1.43±0.25 ms. Somatic recordings were further characterized by the after-hyperpolarization. In most cases, small amounts of negative current were applied to stabilize the membrane potential after penetration. Neuronal data were analysed using Igor pro 6 (Wavemetrics), the software package neuromatic (http:// www.neuromatic.thinkrandom.com ), and custom written scripts (B.P.C.). Spontaneous (s) VOCs, unlike electrically evoked (e) VOCs, lacked electrical artefact and were analysed for both onset and duration of neuronal activity. The duration of sVOCs and eVOCs was measured as the interval between the first and the last VOC waveform, whereas frequency was determined as the quotient of vocal nerve waveform and call duration expressed in Hz (see Fig. 1b ). The variability of the VOC frequency was calculated and expressed as percentage of the average frequency. VPN frequency was calculated for the last four cycles of action potential firing (sustained response) and the first four cycles of prominent subthreshold oscillations ( Fig. 3b ) as the average of the reciprocal of the interval between the minima of two successive cycles (1 per intercycle duration). Instantaneous frequency ( Fig. 3b inset) for the last four cycles of action potential firing and the first eight cycles subthreshold oscillations was the reciprocal of the interval between the minima. Duration of sustained depolarizations in VPP neurons was measured as the half-amplitude width of the depolarization. Peri-event time averages were generated for the sVOC/eVOC and intracellular records using the first VOC waveform as the event trigger. The firing pattern of VPN neurons was visualized using a phase plane plot of the recorded voltage ( V ) against the difference in voltage over time (d V /d t ) for three different excerpts of the same recording: sustained firing, subthreshold oscillations and baseline. The d V /d t trace was smoothed using a Gaussian filter. Statistical analysis was performed with the software JMP. Lidocaine inactivation Micropipettes with diameters of 20–30 μm were fabricated and filled with either 10% lidocaine hydrochloride (Sigma) in 0.1 M PB or 0.1 M PB alone. Baseline and post-injection vocal activity were determined by averaging the eVOC duration (expressed by the number of eVOC waveforms) for 50 consecutive stimulus applications (interstimulus interval of 0.7 s). After baseline recording, the glass micropipettes were stereotactically guided to VPP by surface landmarks and previous mapping studies [27] , [42] . The pipette solution was pressure-ejected using a picospritzer (Biomedical) set to deliver 3 pulses, 10–50 ms duration each, at 25–30 PSI. Bilateral injections were performed sequentially with one micropipette. The eVOCs were monitored and analysed for up to 1 h post injection (recording intervals of 5 min). Typically, one control and one lidocaine injection were made in each animal, with more than a 60 min interval between injections that allowed for complete recovery from any effect of the first injection. The location of injection sites were confirmed in seven cases post hoc using a lidocaine solution (see above) that included 4% fluorescein followed by transcardial perfusion as above (except fixation was only with 3.5% paraformaldehyde in 0.1 M PB) and sectioning of tissue as described earlier. Injection sites were checked using fluorescence microscopy (Nikon Eclipse E800). Pressure injection into VPP of bicuculline, a GABA A receptor antagonist, followed the same method as described above for lidocaine injection. How to cite this article: Chagnaud, B. P. et al . Vocalization frequency and duration are coded in separate hindbrain nuclei. Nat. Commun. 2:346 doi: 10.1038/ncomms1349 (2011).